Efficient AID targeting of switch regions is not sufficient for optimal class switch recombination Antibody affinity maturation relies on activation-induced cytidine deaminase (AID)-dependent somatic hypermutation (SHM) of immunoglobulin (Ig) loci. Class switch recombination (CSR) can in parallel occur between AID-targeted, transcribed, spliced and repetitive switch ( S ) regions. AID thus initiates not only mutations but also double-strand breaks (DSBs). What governs the choice between those two outcomes remains uncertain. Here we explore whether insertion of transcribed intronic S regions in a locus ( Igκ ) strongly recruiting AID is sufficient for efficient CSR. Although strongly targeted by AID and carrying internal deletions, the knocked-in S regions only undergo rare CSR-like events. This model confirms S regions as exquisite SHM targets, extending AID activity far from transcription initiation sites, and shows that such spliced and repetitive AID targets are not sufficient by themselves for CSR. Beyond transcription and AID recruitment, additional IgH elements are thus needed for CSR, restricting this hazardous gene remodelling to IgH loci. Class switch recombination (CSR) occurs at immunoglobulin heavy chain ( IgH ) loci after mature B-cell activation [1] . By changing the IgH chain constant ( C H ) gene, it switches from IgM/IgD production to either IgG, IgA or IgE [2] . At the gene level, CSR needs ‘switch’ ( S ) regions located 5′ of C H genes to undergo double-strand breaks (DSBs), before donor ( Sμ ) and acceptor ( Sγ , Sα or Sɛ ) regions can be joined and bring a downstream C H gene in place of Cμ . CSR and occurrence of DSBs require adequate chromatin structure, looping of IgH loci [3] and transcription of target C H genes within specific units associating a I-promoter, a non-translatable ‘I-exon’, an intronic S region and the coding C H exons [1] . Although its role is still unclear, this germline transcription (GLT) initiating from I -promoters and running through S and C regions is mandatory for CSR and S region accessibility to the activation-induced cytidine deaminase (AID) enzyme [4] . S regions are 1–10 kb-long highly repetitive DNA sequences containing RGYW motifs targeted by AID [5] . AID, also implicated in the somatic hypermutation (SHM) of V(D)J exons, catalyses cytosine (C) deamination into uracyl (U), such lesions being further processed by either the base excision repair (BER) or mismatch repair (MMR) machinery [5] . G-rich S regions may form R-loops during their transcription, allowing accessibility of the non-template strand to the enzymatic activity of AID [6] . While GLT is non-productive due to stop codons in all three reading frames of I -exons, CSR needs I -exon splicing onto C H exons [7] . This might be due to the contribution of the splicing regulator PTBP2 to AID recruitment [8] . Recent evidence also suggested that, during CSR, AID directly recruits MMR and BER factors [2] . Processing of G:U mismatches by either MMR or BER initiates DSBs, then repaired by classical or to a lesser extent alternate non-homologous end joining (c-NHEJ or a-NHEJ, respectively) [9] . Besides the architecture of transcriptional units, a long-standing issue about CSR is the role of IgH cis- regulatory elements. If the intronic Eμ enhancer has only a modest role during CSR [10] , the IgH 3′ RR lying downstream of the last Cα exon, has long been described as a master regulator of CSR and recently appeared as also mandatory for SHM, its complete deletion in mice abrogating both processes [11] , [12] , [13] . The 3′ RR deletion strongly decreases GLT of some C H genes and modestly affects pV H transcription. The nearly complete V H DJ H SHM blockade in 3′ RR -deleted mice, suggests that the 3′ RR also directly helps recruiting AID to V(D)J exons [13] . Whether the 3′ RR also specifically attracts the CSR machinery onto S regions and/or promotes IgH locus bending and S–S synapses remains to be determined. Finally, although it was proposed that staggered single-strand breaks in repetitive S regions can initiate DSBs [14] , it is unclear whether solely the S region structure controls the choice between processing AID attacks into either single-strand lesions and SHM or the occurrence of DSBs followed with long distance deletions. To determine the minimal requirements for the induction of DSBs and CSR, we created a model whereby transcribed S regions were introduced into the Igκ locus normally targeted by SHM. This ‘Knock-In Kappa Switch’ ( KIKS ) mice expressed a functional human Ig Cκ exon ( hCκ ) flanked by two transcribed S regions, downstream of the last Jκ and thus of endogenous rearranged VκJκ exons. Hence, a complete CSR substrate was placed at sites naturally targeted by AID during SHM, while its CSR efficiency could be monitored by following the switch from hCκ to murine Cκ ( mCκ ) expression. Expression of hCκ supported B-cell development in KIKS mice, as previously reported in another mouse featuring hCκ expression [15] . However, despite efficient transcription and AID targeting of S regions, the KIKS locus only displayed minimal CSR in few B cells within Peyer’s patches (PP). This clearly uncouples the two issues of AID attacks, SHM and CSR. It demonstrates the requirement for specific IgH cis -acting elements which, beyond transcription and AID recruitment onto repetitive targets, finally promote efficient CSR at the IgH locus. KIKS locus description and B-cell development in KIKS mice To determine the minimal requirements for the occurrence of DSBs and CSR after AID DNA lesions, we inserted core Sμ and Sγ3 regions within the Igκ locus. These S regions were inserted into the spliced introns of tandem transcriptional units, but with promoter, enhancer and intron sequences from Igκ origin. This strategy avoided any possible influence of IgH cis -acting elements other than S regions on the artificial KIKS locus, although its architecture mimicked the IgH locus, with S regions comprised into the spliced introns of tandem transcriptional units ( Supplementary Fig. 1a ). Thus, transcription of the KIKS donor Sμ was driven by the promoter of the rearranged Vκ, while constitutive transcription of the acceptor Sγ3 was ensured by a second knocked-in pVκ promoter. Sγ3 is also preceded by a small non-coding exon (leader Vκ4–63 with an inserted stop codon but retaining its natural donor splice site) to ensure its splicing onto the mCκ exon and mimic non-productive IgH GLTs ( Fig. 1 ). This strategy also forbids translation of any truncated and potentially harmful mCκ-LC. AID was expected to target the KIKS Sμ since it stands immediately downstream of rearranged VκJκ exons. Regarding the acceptor Sγ3 , insertion of an additional pVκ in the Igκ locus was previously shown to recruit AID [16] . Before any Sμ–Sγ3 recombination, VJ-rearranged KIKS loci encode a chimeric ‘hκ-LC’ combining a murine V with a human C domain. If CSR-like events occur, Sμ–Sγ3 recombination should remove the human Cκ and yield a fully murine κ-LC (mκ-LC; Fig. 1 ). 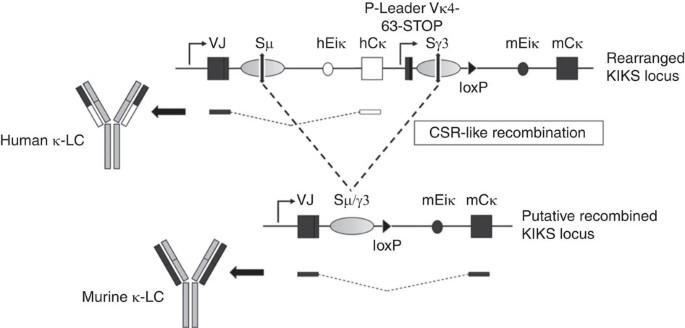Figure 1: Representation and expression of theKIKSlocus. FunctionalKIKS VJrearrangements yield Ig with a humanCκregion.KIKSCSR-like events joinSregions, then excisinghCκand yielding Ig with murineCκ. B-cell development was normal in homozygous KIKS mice regarding bone marrow pro-, pre- and immature B cells and proportions of splenic marginal zone and follicular (Fo) B cells ( Supplementary Table 1 ), with percentage of κ-expressing B cells identical to wild-type (WT) mice ( Supplementary Fig. 1b , left panel). The efficient association of the hκ-LC with murine HC was demonstrated by the similar membrane expression level of IgM and IgD in KIKS compared with WT B cells ( Supplementary Fig. 1b , right panel). KIKS serum κ-LC levels were also similar to WT mice (mean±s.e.m. : 3.72±0.44 versus 4.80±0.45 mg ml −1 , P =0.15, respectively, Supplementary Fig. 1c ). The KIKS Igκ locus thus supports normal B-cell development and function in mice, as observed in another model [15] . Our reporter system was designed to easily monitor CSR-like recombination within the KIKS locus by detecting a switch from human to murine κ-LC at the B-cell surface. In non-immunized KIKS mice, mκ-LC-expressing B cells were below significant detection by flow cytometry ( Supplementary Fig. 1b , right panel). The few cells staining for both human and murine κ-LC never exceeded background levels set in parallel with nonspecific isotype controls ( Supplementary Fig. 1d ). Accordingly, we only noticed minimal amounts of mκ-LC in sera of KIKS mice (0.017±0.004 mg ml −1 ; Supplementary Fig. 1c ). Figure 1: Representation and expression of the KIKS locus. Functional KIKS VJ rearrangements yield Ig with a human Cκ region. KIKS CSR-like events join S regions, then excising hCκ and yielding Ig with murine Cκ . Full size image KIKS locus undergoes low-level CSR-like recombination To increase the probability of CSR events in spleen, we immunized KIKS mice using intraperitoneal injections of sheep red blood cells (SRBC). Eight days after immunization, mice were analysed. As shown in Supplementary Fig. 1e , germinal centre (GC) generation is similar in KIKS and WT mice, demonstrating that mutant B cells efficiently participate to immune responses. However, <0.2% of B cells expressing only mκ-LC were detectable in both KIKS AID +/+ and AID +/− mice ( Fig. 2a ) despite a clear increase of IgG1 and IgG3-switched cells, witnessing parallel efficient CSR at the IgH locus ( Fig. 2b,c ). These results were confirmed in mice analysed 10 days after booster immunization with SRBC ( Fig. 2c ). Finally, weakness of KIKS CSR was emphasized by the minute level of serum mκ-LC yielded on immunization as compared with IgG1 and IgG3 ( Fig. 2d ). We then analysed PP known to abundantly switch to IgA ( Supplementary Fig. 2a ). A small but significant proportion of these PP B cells was consistently found to express murine κ-LC (0.68±0.09% in KIKS AID +/+ and 0.63±0.13% in KIKS AID +/− mice, mean±s.e.m. ; Fig. 2c,e ), a population specifically enriched among GC B cells ( Fig. 2e , lower panel). AID dependence of these CSR-like events was confirmed by their absence in AID-deficient KIKS mice ( Fig. 2c,e ). Finally, we induced CSR in KIKS B cells by 4 days in vitro stimulation. Cytometry analysis indicated that, despite normal IgG3 and IgG1 CSR, the percentage of mκ-LC-expressing cells still remained extremely low (0.37±0.05% and 0.40±0.04%, mean±s.e.m., after lipopolysaccharide (LPS) or anti-CD40+IL-4 stimulation, respectively) albeit significantly higher than in AID −/− stimulated B cells ( Supplementary Fig. 2b ). Altogether, these data show that the KIKS locus can undergo CSR-like events but only at a low level and in conditions only achieved on strong B-cell stimulation, such as in mucosae-associated lymphoid tissues. 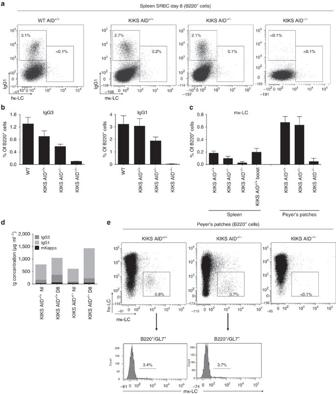Figure 2: Low level of CSR-like recombination inKIKSmice. (a) Representative flow cytometry analyses of CSR in spleen B cells (B220+) from SRBC-immunized mice. Percentages of B cells expressing IgG1 or murine κ-LC are indicated. (b) Comparison ofIgHCSR efficiency in WT,KIKS AID+/+,KIKS AID+/−andKIKS AID−/−mice on SRBC immunization. Percentages of switched B cells in spleen are shown (mean±s.e.m.) (c) Comparison ofKIKSCSR efficiency inKIKS AID+/+,KIKS AID+/−andKIKS AID−/−mice on SRBC immunization (days 8 and 10 after boost). Percentages of mκ-LC switched B cells in spleen and PP are shown (mean±s.e.m.). Forb,c,n=6 mice of each strain except forKIKS AID−/−,n=4 mice in at least two independent experiments. (d) ELISA quantification of serum mκ-LC (black) as compared with IgG1 (light grey) and IgG3 (dark grey) in non-immunized (NI) and SRBC-immunized mice. Superimposed means (μg ml−1) are shown (n=4–6 mice per group in two independent experiments).(e) Representative flow cytometry analyses of human and mouse κ-LC expression among B220+cells in PP ofKIKS AID+/+,KIKS AID+/−andKIKS AID−/−mice. Percentage of mκ-LC+on total B cells (B220+) (upper panel) and on GC B cells (B220+GL7+) is represented (bottom panel). Figure 2: Low level of CSR-like recombination in KIKS mice. ( a ) Representative flow cytometry analyses of CSR in spleen B cells (B220 + ) from SRBC-immunized mice. Percentages of B cells expressing IgG1 or murine κ-LC are indicated. ( b ) Comparison of IgH CSR efficiency in WT, KIKS AID +/+ , KIKS AID +/− and KIKS AID −/− mice on SRBC immunization. Percentages of switched B cells in spleen are shown (mean±s.e.m.) ( c ) Comparison of KIKS CSR efficiency in KIKS AID +/+ , KIKS AID +/− and KIKS AID −/− mice on SRBC immunization (days 8 and 10 after boost). Percentages of mκ-LC switched B cells in spleen and PP are shown (mean±s.e.m.). For b , c , n =6 mice of each strain except for KIKS AID −/− , n =4 mice in at least two independent experiments. ( d ) ELISA quantification of serum mκ-LC (black) as compared with IgG1 (light grey) and IgG3 (dark grey) in non-immunized (NI) and SRBC-immunized mice. Superimposed means (μg ml −1 ) are shown ( n =4–6 mice per group in two independent experiments). ( e ) Representative flow cytometry analyses of human and mouse κ-LC expression among B220 + cells in PP of KIKS AID +/+ , KIKS AID +/− and KIKS AID −/− mice. Percentage of mκ-LC + on total B cells (B220 + ) (upper panel) and on GC B cells (B220 + GL7 + ) is represented (bottom panel). Full size image Knocked-in switch regions are involved in CSR-like events To further confirm that the few B cells expressing mκ-LC carried CSR-like recombination, Sμ/Sγ3 junctions were cloned and sequenced from in vitro -stimulated B cells (LPS and CD40+IL4) and PP cells. Nested PCR primers amplified genomic DNA from the Jκ5 exon to the 5′ part of the loxP site ( Supplementary Fig. 3a,b ), and yielded bands in PP cells from KIKS AID +/+ and AID +/− mice but not from KIKS AID −/− cells or stimulated B cells ( Supplementary Fig. 3c ). We then cloned the amplified bands, which indeed corresponded to junctions of break points located within or close to Sμ and Sγ3 . Locations of break points are depicted on Fig. 3a and junction sequences are shown in Supplementary Fig. 4 . Strikingly, Sμ and Sγ3 sequences around junctions carried very high mutation loads of 33.5 and 25.3 mutations per kb, respectively ( Fig. 3b ). Junctions involved essentially direct joins or short microhomologies (≤3 nt), with no apparent bias toward A-NHEJ ( Fig. 3c ). In conclusion, CSR-like events occurred at low level in the KIKS S regions but associated with intense local AID recruitment and SHM levels far above those usually reported around normal IgH S -junctions [17] . 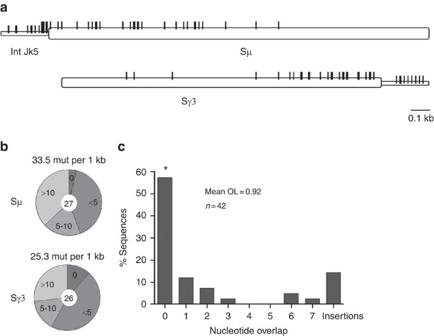Figure 3: Analysis ofKIKSCSR-like junctions. (a) Location of DNA breaks (vertical lines) inSμor intronJκ5(Int Jκ5) (top) andSγ3(bottom) implicated in each sequenced junction. (b) Mutation rates (mutation per kb) in joinedSμ(top) andSγ3(bottom) are indicated above the pie charts. Segment sizes in the pie charts are proportional to the number of sequences carrying the number of mutations indicated in the charts. The number of independent sequences analysed is indicated in the centre of each chart. (c) Analysis of microhomology atSμ/Sγ3junctions inKIKSGC B cells. Histograms represent the percentage ofSμ/Sγ3junction sequences with indicated nucleotide overlap. Mean length of overlap in base pairs (OL) and number of sequences analysed (n) are indicated. * Sequences with small insertions (one to three nucleotides) at the junction were scored as zero microhomology and represent 15% of total junctions. Forb,c, results were obtained from four independent experiments in which PP of three mice were pooled. Figure 3: Analysis of KIKS CSR-like junctions. ( a ) Location of DNA breaks (vertical lines) in Sμ or intron Jκ5 ( Int Jκ5 ) (top) and Sγ3 (bottom) implicated in each sequenced junction. ( b ) Mutation rates (mutation per kb) in joined Sμ (top) and Sγ3 (bottom) are indicated above the pie charts. Segment sizes in the pie charts are proportional to the number of sequences carrying the number of mutations indicated in the charts. The number of independent sequences analysed is indicated in the centre of each chart. ( c ) Analysis of microhomology at Sμ/Sγ3 junctions in KIKS GC B cells. Histograms represent the percentage of Sμ/Sγ3 junction sequences with indicated nucleotide overlap. Mean length of overlap in base pairs (OL) and number of sequences analysed ( n ) are indicated. * Sequences with small insertions (one to three nucleotides) at the junction were scored as zero microhomology and represent 15% of total junctions. For b , c , results were obtained from four independent experiments in which PP of three mice were pooled. Full size image Knocked-in switch regions of KIKS are accessible to AID Scarcity of KIKS CSR-like recombination could have reflected poor AID recruitment on the knocked-in Sμ and/or Sγ3 . As AID targeting of S regions needs transcription, we checked the transcriptional activity at inserted S regions. It can obviously be inferred from the normal level of hκ-LC expression in KIKS B cells that Sμ is efficiently transcribed and spliced out. Likewise, we also readily detected LVκ4–63/mCκ transcripts implying transcription and splicing of the inserted Sγ3 ( Supplementary Fig. 5b ). To more specifically address the transcriptional abundance of KIKS S regions, we carried out quantitative PCR on primary transcripts of both KIKS Sμ and Sγ3 . We observed about fivefold less Sγ3 transcripts compared with Sμ , a difference comparable to that obtained at the IgH locus in LPS-stimulated B cells, a condition known to efficiently induce Iγ3 transcription and CSR to IgG3 (ref. 12 ; Supplementary Fig. 5b ). Since both S regions are transcribed in a locus naturally accessible to AID, we checked the mutation frequencies within Sμ and Sγ3 before CSR. For Sμ , we analysed 570 bp downstream Jκ5 , comprising 220 bp from the Jκ intron and 350 bp from the inserted Sμ ( Fig. 4a ). As mutations occur within a range of 1.5 kb after the V promoter, with a rate decreasing with promoter distance and highest in the VJ exon, we checked if this distance also affected SHM in Sμ and compared KIKS Sμ mutations following rearrangement of either distant ( Jκ1 ) or proximal ( Jκ5 ) VκJκ rearrangement ( Fig. 4a ). For Sγ3 , we analysed the first 400 bp ( Fig. 4b ). As expected, mutation frequencies within the knocked-in Sμ and Sγ3 were far higher in sorted PNA high Fas + GC B cells than in resting KIKS AID +/+ PPs B cells ( Fig. 4a,b and Table 1 ). VJκ5 -rearranged alleles revealed similar SHM frequencies in Jκ5 intron and in Sμ (11.19 versus 13.08 mutations per kb). This is consistent with data reported in the equivalent region of the WT Igκ locus [13] , [18] . Surprisingly, VJκ1 -rearranged KIKS loci also revealed high SHM rates within the knocked-in Sμ (7.80 mutations per kb; Table 1 ) although it lies more than 2 kb downstream of pVκ , that is, at a distance normally escaping mutations downstream of rearranged VJ exons [19] ( Fig. 4a ). This high mutation rate at long distances from the promoter likely involved an increased and/or extended AID recruitment on S sequences containing highly repetitive RGYW motifs, as recently demonstrated for Sγ1 (ref. 20 ). However, a similarly frequent SHM affected the Jκ5 intron from the same rearranged loci (8.10 mutations per kb). To exclude any local effect due to the close proximity of Sμ , analyses were extended upstream of Jκ5 in a region lying from ∼ 1.3 to 1.8 kb downstream of pVκ ( Jκ3 ) thus supposed to mostly escape SHM [19] (primer 9, Supplementary Fig. 3 ). Here again, high SHM occurred in GC B cells, reaching 11.17 mutations per kp ( Table 1 ). The knocked-in Sγ3 from GC B cells also carried high SHM at 7.30 mutations per kb ( Fig. 4b and Table 1 ), that is, slightly lower than for Sμ lying on VJκ5 KIKS alleles at an equivalent distance from a pVκ , but clearly higher than reported for IgH Sμ in WT GC B cells undergoing CSR (4.10 mutations per kp; Fig. 4c and Table 1 ) or in vitro [13] , [21] , [22] , [23] . Chromatin immunoprecipitation (ChIP) analysis also showed the accumulation at KIKS S regions of acetylated histone H3K9 (H3K9ac), a chromatin mark known to be associated with the transcriptional activity and accessibility of S regions allowing AID recruitment and activity ( Supplementary Fig. 6 , top panel) [24] , [25] . Thus, the KIKS S regions are strongly targeted by AID and SHM, although this is clearly not followed with efficient CSR. 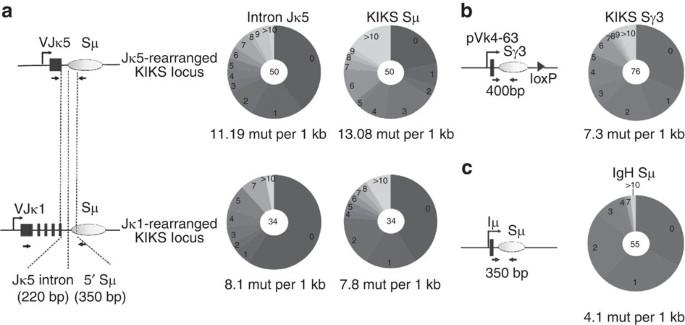Figure 4:KIKSlocus is accessible to AID. (a) Analysis of mutations inKIKS Sμregion according toVJrearrangement. Left panel: the two primers used for amplification (short arrows) allow amplification ofKIKSalleles that are rearranged to all theJκsegments but analyses were carried out onJκ5(top) orJκ1(bottom) rearrangements. For bothJκ5andJκ1rearrangements,Jκ5intron and 5′ part ofSμregion were sequenced. Right panel: pie charts analyses ofJκ5intron and 5′Sμmutations from sorted GC (B220+PNAhighFas+) PP B cells fromKIKSmice. Segment sizes of the pie charts are proportional to the number of sequences bearing the indicated numbers of mutations. Numbers of analysed sequences (centre of pie charts) and number of mutations per kb (mut per kb) are indicated (below pie charts). (b) Analysis of mutations inKIKS5′Sγ3region from the same cells as ina. Sequenced region, amplified with indicated primers (shorts arrows), is represented. Pie chart features are the same than ina. (c) Analysis of mutations inIgH Sμregion from the same cells as ina. Sequenced region, amplified with indicated primers (shorts arrows) is represented. Pie chart features are the same than ina. Figure 4: KIKS locus is accessible to AID. ( a ) Analysis of mutations in KIKS Sμ region according to VJ rearrangement. Left panel: the two primers used for amplification (short arrows) allow amplification of KIKS alleles that are rearranged to all the Jκ segments but analyses were carried out on Jκ5 (top) or Jκ1 (bottom) rearrangements. For both Jκ5 and Jκ1 rearrangements, Jκ5 intron and 5′ part of Sμ region were sequenced. Right panel: pie charts analyses of Jκ5 intron and 5′ Sμ mutations from sorted GC (B220 + PNA high Fas + ) PP B cells from KIKS mice. Segment sizes of the pie charts are proportional to the number of sequences bearing the indicated numbers of mutations. Numbers of analysed sequences (centre of pie charts) and number of mutations per kb (mut per kb) are indicated (below pie charts). ( b ) Analysis of mutations in KIKS 5′ Sγ3 region from the same cells as in a . Sequenced region, amplified with indicated primers (shorts arrows), is represented. Pie chart features are the same than in a . ( c ) Analysis of mutations in IgH Sμ region from the same cells as in a . Sequenced region, amplified with indicated primers (shorts arrows) is represented. Pie chart features are the same than in a . Full size image Table 1 Analysis of mutations in KIKS and IgH loci in Peyer’s patches B cells. Full size table DSBs occur in KIKS S regions Given that KIKS S regions are efficiently targeted by AID, CSR-like events scarcity could be due to either low occurrence of DSBs and/or their inefficient repair. To address this issue, internal S deletions (ISDs) witnessing resolved DSBs were appreciated within KIKS sequences. Interestingly, such deletions were readily detected in both KIKS S regions, at higher rates than in the corresponding endogenous Sμ region and Jκ5 intron (0.230 and 0.263 ISD per kb in Sμ and Sγ3 regions, respectively, versus 0.054 in endogenous Sμ and 0.037 in non- S regions; Fig. 5a ). The length of ISDs ranged from 16 to 160 bp, obviously biased by the preferential PCR amplification of short ISDs. The KIKS locus thus clearly undergoes AID-initiated DSBs that are proportional to SHM but only in G-rich sequences, consistent with the concept that S regions form R-loops targeted by AID on both the template and non-template DNA strands that hence end with staggered DSBs [6] , [14] . Most of KIKS ISDs display blunt-end junctions or short microhomology and therefore likely result from c-NHEJ repair of DSBs ( Fig. 5b and Supplementary Fig. 7 ). Accordingly, ChIP experiments conducted at the KIKS locus and compared with IgH locus demonstrated the presence of 53BP1, known to protect DNA ends from resection ( Supplementary Fig. 6 , bottom panel) [26] . Finally, since γH2AX was supposed to be dispensable for intraswitch recombination but required for the chromatin remodelling that facilitates distant S region synapsis [23] , we further searched for γH2AX foci associated with the KIKS locus. Immunofluorescence staining followed by fluorescence in situ hybridization (3D immuno-FISH) simultaneously visualized γH2AX and IgH or Igκ loci in GL7 + sorted PP B cells. γH2AX foci associated with Igκ loci at frequencies close to IgH (6.8 versus 8.9%, respectively) confirming the presence of DSBs and their normal initial processing through γH2AX recruitment ( Fig. 5c,d ). 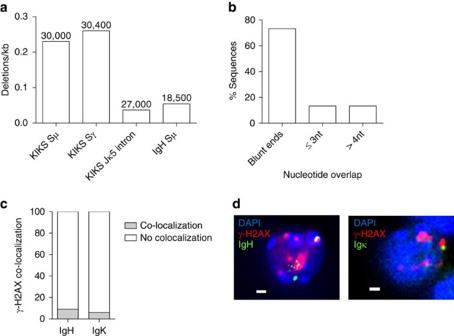Figure 5: DSBs occur normally inKIKSS regions. (a) The number of deletions per kb in switch regions is shown at theKIKSandIgHloci inKIKSmice. Total number of analysed nucleotides is indicated on top of each bars. (b) Analysis of microhomology at total ISD junctions inKIKSGC B cells. Histogram represents the percentage of junction sequences with indicated nucleotide overlap. Fora,b, the number of experiments is the same as inFig. 3. (c) γ-H2AX association withIgHorIgκinKIKSGC B cells. Histogram represents the combination of three independent experiments (individual data set are comparable). ThePvalue calculated with a Fisher exact test is non-significant (P=0.46). (d) Representative images of colocalization between γ-H2AX (red) withIgHlocus (green, left panel) or withIgκlocus (green, right panel). Scale bar, 1 μm. Figure 5: DSBs occur normally in KIKS S regions. ( a ) The number of deletions per kb in switch regions is shown at the KIKS and IgH loci in KIKS mice. Total number of analysed nucleotides is indicated on top of each bars. ( b ) Analysis of microhomology at total ISD junctions in KIKS GC B cells. Histogram represents the percentage of junction sequences with indicated nucleotide overlap. For a , b , the number of experiments is the same as in Fig. 3 . ( c ) γ-H2AX association with IgH or Igκ in KIKS GC B cells. Histogram represents the combination of three independent experiments (individual data set are comparable). The P value calculated with a Fisher exact test is non-significant ( P =0.46). ( d ) Representative images of colocalization between γ-H2AX (red) with IgH locus (green, left panel) or with Igκ locus (green, right panel). Scale bar, 1 μm. Full size image This study addresses the long-standing issue of minimal requirements for CSR versus SHM, two processes sharing several common prerequisites but yielding drastically different genomic and cellular changes. In the IgH locus, S regions susceptible to multiple AID attacks on both DNA strands are mandatory targets for CSR and it is unclear whether other cis -elements of the locus play a role in orienting the processing of AID lesions towards DSBs and/or distant S–S recombination rather than SHM. The aim of our study was thus to check whether two transcribed and spliced S regions located at a position highly recruiting AID, would be sufficient for mediating CSR-like events and being joined at a high level in activated B cells. This issue was addressed in an in vivo model by generating KIKS mice, which carried S regions inserted into the Igκ locus naturally targeted by AID, without any other regulatory element from the IgH locus. By designing the knock-in so that CSR-like events would change LC expression, we observed by flow cytometry that, despite their efficient transcription and splicing-out, the inserted S regions underwent only rare recombination and junction events, even in B cells undergoing high-rate CSR in the IgH locus. Since AID levels are relevant to CSR efficiency [27] , we cannot totally rule out the possibility that additional transcribed S regions could dilute AID activity and then diminish CSR efficiency at the KIKS locus. However and contrary to the herein reported observations, such a sink effect would be expected on one hand to impact both KIKS and IgH CSR, and on the other hand to be more severe in AID +/− mice with half-dose of AID. Moreover, inserted Sγ3 and Sμ regions were mutated in AID-expressing cells, and even both showed mutation rates far above the endogenous Sμ region of B cells undergoing CSR in vitro or in vivo [13] , [21] , [22] , [23] , [26] , [28] . Altogether, this argues against the hypothesis of a sink effect resulting in a local purely quantitative defect of AID in the presence of increased number of target regions. Our data demonstrated that AID and the BER and MMR machineries, all common actors of both SHM and CSR, were highly recruited to the inserted core S regions. A striking finding is the unexpected high mutation rates in both the Jκ5 intron and flanking Sμ region regardless of their distance from the promoter [19] . While Igκ locus enhancers are likely responsible for AID recruitment onto both promoters of the KIKS locus, the extended SHM shows that the inserted S region structure per se modulates the pattern of AID recruitment. These results are reminiscent to the robust AID targeting recently reported in a model in which the core Sγ1 region was inserted in the Bcl6 locus [20] . Thus, tethering of AID appears as an intrinsic property of transcribed S regions. However, by contrast to the Bcl6 model where regions flanking the core Sγ1 were free of AID targeting [20] , we found a sustained high SHM rate throughout the 2-kb-long Jκ region that cannot be fully related to the fact that Igκ is a much better AID target than Bcl6 (ref. 29 ). In the KIKS model, the VJ gene close to the pVκ is initially subjected to SHM and it is likely that the distal G-rich S region not only recruits but also maintains AID tethering throughout the entire transcribed Jκ region as it certainly processes in the IgH locus to target the whole extent of S regions on distances up to 10 kb (ref. 25 ). In current models of CSR, richness of core S regions in RGYW motifs is claimed to allow the generation by AID and UNG of staggered DSBs then recruiting the NHEJ machinery [2] . Accordingly, γH2AX foci are readily detected at KIKS loci together with short ISDs in KIKS S regions at higher rates than in the IgH Sμ (likely related to the locally increased SHM), confirming the occurrence of DSBs and their repair with no bias towards A-NHEJ. We also readily detected 53BP1 recruitment in the KIKS S regions, further indicating that DNA ends are likely protected from resection and overwhelmingly repaired by classical NHEJ similar to normal IgH S region DSBs [26] . Altogether, these ISDs demonstrate that, besides high AID targeting indicated by SHM, DSBs are also generated and normally processed into KIKS S regions. Therefore, the poor ability of the KIKS locus to undergo CSR most likely reflects a defect in synapsis between the distant Sμ and Sγ3 and/or their inefficient recruitment into ‘CSR factories’ supporting recombination at long distance. This deserves comparison with recent studies showing that distant DSBs induced by high efficiency endonucleases (I-SceI meganuclease or Crispr/Cas9) are efficiently processed through a general cis -joining mechanism needing neither local transcription nor specific chromosomal localization, provided that they are comprised within the 1-Mb spreading range of the γH2AX-dependent DNA damage response [26] , [28] , [30] . Although such models interestingly underlined that any cell can efficiently handle distant DSBs in cis , it differed from CSR by multiple features. According to the DNA deamination model, CSR uses no endonuclease directly generating DSBs but rather needs processing of single-strand DNA bubbles appearing around mismatches. Together with the low SHM observed in S regions of GC B cells, it is then tempting to speculate that, by contrast to endonuclease-induced DSBs, the occurrence of two synchronous distant AID-induced DNA breaks should be rare in physiology, needing recruitment in specialized CSR factories to be efficiently joined and repaired. In addition, I-Sce-I-induced DSBs underwent extensive end processing [28] , a condition rarely encountered during AID-induced CSR at the IgH or KIKS loci in which blunt ends are essentially processed through c-NHEJ, thus preserving locus integrity. In fact, AID remodelling of the KIKS locus resembles models of ‘failed’ CSR-like 53BP1 −/− , γH2AX −/− or AID carboxyl-terminal region mutants, with normal SHM and intraswitch region recombination but only rare CSR junctions between distant S regions [23] , [26] , [31] . While such defects of the potential ‘CSR factory’ components are absent in our model (where normal IgH CSR occurs), the KIKS locus might then simply demonstrate a defective recruitment of the knocked-in S regions into such CSR factories. Whether the Igκ locus may intrinsically dictates differential outcome of AID-induced lesions, as it was recently demonstrated when S regions were knocked-in in other loci [20] , [32] , is another possibility. But the presence of ISDs, few S-S junctions, 53BP1 recruitment and γH2AX foci, proves that beside AID-induced single-strand mutations, DSBs occur at the KIKS locus but are not appropriately handled for efficient synapsis and junction of distant breaks. We thus propose that beside the general possibility for DSBs to be cis -joined over long distances, optimal CSR requires additional IgH cis -regulatory elements recruiting and synapsing target regions into specific nuclear areas with the functional ability to coordinate and associate distant DSBs and promote long-range recombination. Hereby constraining CSR to the IgH locus would also help prevent side genomic alterations. In this view, it would be relevant to check if the presence of S regions outside of their physiological loci could increase, as previously described in c-Myc [32] , translocation potential and genomic instability in KIKS cells and to what extent. This work brings new insights in the molecular dissection of CSR. It demonstrates in a locus physiologically targeted by AID, that transcription, splicing, efficient SHM and occurrence of DSBs repairs by c-NHEJ into S regions are not sufficient to trigger CSR. We thus propose that the early events of CSR from cytidine deamination to occurrence of DSBs can affect any G-rich transcribed and spliced genomic position targeted by AID. By contrast, only the IgH locus context provides all the additional conditions for long-range synapsis between AID targets and efficient CSR. A good candidate for assembling the latter conditions is obviously the 3′ RR , as its deletion in mouse drastically impairs CSR and was also shown to impair IgH synapsis [12] . Long-range interactions between IgH 3′ RR , Eμ and I -promoter activated by specific stimulation, was shown to allow the acceptor S region to interact with Sμ , then contributing to the stability of S–S synapsis during CSR [33] . Since 3′ RR deletions globally affected IgH SHM, GLT and CSR, its complex functions can hardly be analysed by knockout experiments. Whether the sole downregulation of GLT or the concomitant lack of synapsis-promoting elements explains the lack of CSR in 3′ RR mutant mice remains to be addressed. The adjunction of the 3′ RR to the KIKS locus could provide insight into this issue. Others potential regulators of CSR are I -promoters that drive acceptor S region transcription before CSR and could participate in recruiting CSR factors [3] . Finally, we also cannot fully rule out the possibility that the KIKS S regions are too close to each other to allow optimal looping of the chromosome during synapse. While further investigations are needed to decipher the exact contribution of each of these elements, the KIKS strategy already sheds new light on the minimal requirements for efficient CSR, that are clearly beyond transcription, AID recruitment and occurrence of DSBs. Generation of KIKS mice The previously described 12.7 kb Bam HI fragment from the Igκ locus containing the 5 Jκ segments and Cκ was used [34] . The 0.8-kb Bst EII fragment, located 0.2 kb downstream of Jκ5 was eliminated and replaced by a NotI site, then allowing the sequential cloning of the fragments composing the KIKS locus using EagI and NotI compatible sites. Sμ region comprises a HindIII 1.9 kb fragment from a plasmid containing the murine JH-Cμ region [35] with 1.5 kb of core Sμ repeats. A 2-kb fragment of the Sγ3 sequence (Genebank accession number M12182 ) was amplified from C57BL/6 genomic DNA, with the indicated primers ( Supplementary Fig. 3b ), and features the entire repetitive region, previously described [36] . Equivalent S regions were previously shown to efficiently support CSR in several studies [37] , [38] , [39] . From 5′ to 3′, the following parts were then added: the murine core Sμ , a 1.5-kb genomic fragment containing human Eiκ and Cκ , a 0.3-kb fragment containing Vκ4–63 promoter and the following leader exon (in which the last codon was replaced by a stop codon to mimic a non-translatable I-exon) and the murine core Sγ3 . A neomycin-resistance gene ( Neo R ) flanked with two loxP sites was inserted downstream Sγ3 . Upstream of the 5′ arm, a thymidine kinase ( TK ) gene was inserted for negative selection against random integration. E14 embryonic stem cells were transfected with linearized vector and selected by addition of G418 and ganciclovir to culture medium. An embryonic stem clone showing homologous recombination of the Igκ locus by Southern blot was injected into C57BL/6 blastocysts, and resulting chimeras were mated with C57BL/6 animals. Progeny was then bred with EIIa-CRE mice (a gift from Dr H. Westphal, Bethesda, MD) to obtain a Neo R -deleted KIKS lineage and avoid any transcriptional competition from the Neo R promoter. Mice were first screened by PCR for the presence of the human Cκ exon and then for homozygous loss of the WT allele. All the animal strains were bred and maintained in pathogen-free conditions and analysed at 8–16 weeks of age. All the protocols used have been approved by our institutional review board for animal experimentation (Comité Régional d’Ethique de l’Expérimentation Animale du Limousin). Sample size was determined to support statistical analysis while minimizing the number of animals involved. No animal was excluded from the analysis. Immunization and spleen cell cultures Mice were immunized by intraperitoneal injection of 200 μl of SRBC and analysed after 8 days. In some cases, mice were booster immunized at day 20 with a second injection of 100 μl of SRBC and analysed 10 days after. Total spleen cells were cultured at a density of 1 × 10 6 cells ml −1 in RPMI 1640 supplemented with 10% fetal calf serum either with 50 ng ml −1 LPS (Sigma-Aldrich, St Quentin Fallavier, France), alone or plus 20 ng ml −1 IL4 (PeproTech, Rochy Hill, NJ) or IL4 plus 5 μg ml −1 anti-CD40 (R&D Systems, Minneapolis, MN). Flow cytometry and cell sorting Antibodies and reagents used for staining and cell sorting experiments are detailed in Supplementary Table 2 . Flow cytometry analyses were done on a BD Pharmingen LSRFortessa cytometer. Data were then analysed with BD FACSDiva software (BD Biosciences, San Jose, CA). Intracellular staining for flow cytometry was done using BD Cytofix/Cytoperm Kit following the manufacturer’s instructions (BD Biosciences). For SHM analyses, GC (B220 + /PNA high /Fas + ) and resting (B220 + /PNA low /Fas − ) B cells from PP were sorted. Cell sorting experiments were done on a BD Pharmingen FACSVantage cell analyser. SHM and S-junction analyses Genomic DNA from total PP cells ( S -junctions) or sorted B-cell subsets was extracted using standard proteinase K procedures. All DNA sequences for SHM were amplified using Phusion high-fidelity DNA polymerase (New England BioLabs) with primers indicated in Supplementary Fig. 3 , cloned into pGEM-T Easy vector (Promega, Madison, WI), sequenced with the BigDye Terminator kit on a 3130xl Genetic Analyzer (Applied Biosystems) and analysed using Finch TV software. Mutations were counted for each sequence, then added and divided by the total number of analysed nucleotides to obtain mutation frequency. For junction analysis, DNA was subjected to two rounds of PCR with nested primers ( Supplementary Fig. 3 ). The first round of PCR consisted in 10 cycles followed by a second round of 32 cycles. ELISA assays Human and mouse κ light chains, IgG1 and IgG3 in sera from WT and KIKS mice were evaluated by ELISA (enzyme-linked immunosorbent assay) as previously described [40] . In brief, 96 multiwell plates (Maxisorb, Nunc, Denmark) were coated overnight with 1 μg ml −1 with appropriate antibodies ( Supplementary Table 2 ) in NaHCO 3 buffer. Plates were then blocked with PBS containing 3% bovine serum albumin for 30 min and diluted sera samples or standards were incubated for 2 h at 37 °C. Alkaline phosphatase-conjugated antibodies were incubated for 1 h 30 at 37 °C and followed by the addition of p -Nitrophenyl phosphate (Sigma-Aldrich). Reading of plates was done at 405 nm with a SAFAS Xenius device. Transcript analysis Total RNA from PP was extracted with TRI Reagent (Ambion, Austin, TX), according to the manufacturer’s protocol, and 1 μg was used for cDNA synthesis using hexameres (Applied Biosystems). End-point PCR of mature transcripts was performed using Q-biogen Taq polymerase (Qiagen). Relative quantification of primary transcripts was performed with SYBR green Master Mix (Applied Biosystems) and compared with GADPH levels. Primers are indicated in Supplementary Fig. 3 . Immuno-FISH 3D GC B cells (GL7 + ) from murine PP were dropped onto poly- L -lysine slides and fixed with 2% paraformaldehyde for 10 min at room temperature. After washing with PBS, cells were permeabilized with 1% Triton-X-100 for 15 min at room temperature. Cells were stained with γ-H2AX antibody (1/300, Millipore) overnight at 4 °C followed by secondary goat anti mouse IgG (1/1000, Invitrogen) during 1 h at room temperature. After three washes with PBS/Tween 0.1%, cells were postfixed in 2% paraformaldehyde for 10 min at room temperature and permeabilized with Triton-X-100 1% HCl 0.1 M for 20 min at room temperature. Denaturation was performed during 35 min with 2 M HCl at room temperature and slides were rinsed three times in cold PBS. Cells were hybridized overnight at 37 °C with IgH (5′ IgH ) or Igκ (RP23–341D5) probes labelled with dUTP-digoxigenine (Roche). The next day, cells were washed in 1 × saline sodium citrate (SSC) at 72 °C for 5 min and 1 × SSC at room temperature for 5 min. Then, the cells were incubated with anti-digoxigenine FITC (1/300, Abcam) 1 h at room temperature and washed three times in 2 × SSC. Finally, the slides were mounted with vectashield (Vector labs). Images were acquired with an epifluorescence inverted microscope (LEICA DMI6000B). Optical sections separated by 0.2 μm were collected and stacks were deconvoluted using Huygens software and analysed with Image J software. Chromatin immunoprecipitation We used the ChIP-IT Express Kit (Active Motif) according to the manufacturer’s instructions. In brief, 5 × 10 6 PP cells were fixed with 1% formaldehyde at room temperature. The reaction was stopped by adding glycine to a final concentration of 0.125 M. After the crosslinking reaction, cell lysis and sonication were performed on Vibracell sonicator (Sonics and Materials, Inc). For immunoprecipitation, 4 μg of each antibody was added to the lysate at 4 °C overnight. The immunoprecipitated DNA was used for real-time PCR using SYBR Green Master Mix (Applied Biosystems). The quantitative PCR signal was normalized using the % input method. Primers for KIKS locus are listed in Supplementary Fig. 3 (or as in Wang et al . [25] for the IgH locus). Antibodies used for pull down of DNA associated with H3K9Ac and 53BP1 or negative control antibody (Millipore) are indicated in the Supplementary Table 2 and were previously described [25] , [41] . Statistical analysis The statistical tests used to evaluate differences between variables were indicated in legends and were done using Prism GraphPad software (San Diego, CA). All P values <0.05 were considered significant. How to cite this article: Bonaud, A. et al . Efficient AID targeting of switch regions is not sufficient for optimal class switch recombination. Nat. Commun. 6:7613 doi: 10.1038/ncomms8613 (2015).